Seismic detection of increased degassing before Kīlauea's 2008 summit explosion Monitoring of active volcanoes is best accomplished by using a variety of geophysical, geochemical and geological data sets to unravel the complex processes that precede and accompany unrest. Seismology is at the core of such monitoring efforts, given the close association between eruptions and seismicity [1] , and it is often the only technique available when resources are sparse. To best take advantage of the limited data available at many volcanoes, it is therefore important to develop methods of analysis that link seismic observations to temporally variable volcanic processes [2] . Seismic data are used to identify the occurrences, locations and styles of earthquakes, but also provide information beyond these traditional measures. For example, the height of ash columns during explosive eruptions can be inferred by combining seismic amplitudes with eruption column models [2] . When three-component seismic stations are available, it is possible to measure the directional properties of earthquake waves (seismic anisotropy) that vary in the crust according to alignment of minerals or microcracks, the nature of the fluids in the cracks and the presence of layering or fractures (for example, Zinke and Zoback [3] , Keir et al [4] and Boness and Zoback [5] ). A shear wave in an anisotropic medium will be split into a fast and a slow velocity component, with fast wave orientation ϕ and delay time between the two waves δ t . The measurement of seismic anisotropy using the method of shear wave splitting (SWS) has been found to be a proxy for determining the direction of maximum horizontal compressive stress in the crust [5] ; applied stress can cause microcracks to preferentially open parallel to the maximum compressive stress, creating an anisotropic medium with the fast direction parallel to the maximum horizontal compressive stress [6] . The mechanism of aligned microcracks is thought to be the only one that allows seismic anisotropy to vary on observable time scales [7] , and temporal changes are traditionally interpreted as stemming from variations in the stress field due to large earthquakes [7] or magmatic intrusions [8] . There is mounting evidence, however, that the dominant mechanism for SWS can switch between a static condition, such as aligned fractures in fault zones, and a dynamic process, such as maximum horizontal compressive stress causing aligned microcracks to dilate [9] , [10] . In areas where there are strong changes in maximum compressive stress direction and magnitude on observable timescales, such as at active volcanoes, SWS analysis has proven a valuable tool when combined with ground deformation or other seismological observations for interpretation of volcanic processes such as magma migration [8] , [9] , [10] , [11] , [12] , [13] . Such changes are always detected in hindsight, however, and seismologists struggle to employ monitoring of seismic anisotropy in real- or near-real-time to assist in eruption forecasting. By applying SWS at well-monitored, highly active volcanoes, like Kīlauea, it may be possible to connect changes in seismic anisotropy to specific volcanic processes, such as volcanic degassing. We found that the orientation of fast shear waves at Kīlauea is usually controlled by structure, but in 2008 showed changes with increased SO 2 emissions preceding the start of the summit eruption. Combining SWS with V p / V s data allowed us to conclude that the changes were due to increased gas-filled pore pressure. This knowledge is critical to enhancing our ability to monitor under-instrumented volcanoes. SWS fast orientations We have performed SWS analysis at the summit of Kīlauea Volcano on 2,168 local earthquakes with M l ≥ 2 recorded at 10 three-component seismic stations ( Fig. 1 ) from the beginning of 2007 until the end of 2011, achieving 8,359 reliable measurements (see Methods section for selection criteria and quality-control steps). The time period spans the onset of Kīlauea's currently ongoing summit eruption, which began on 19 March 2008 [14] , [15] . Figure 2 displays the fast orientation of SWS ( ϕ ) as rose diagrams at the station where the recording was made for each year between 2007 and 2011. 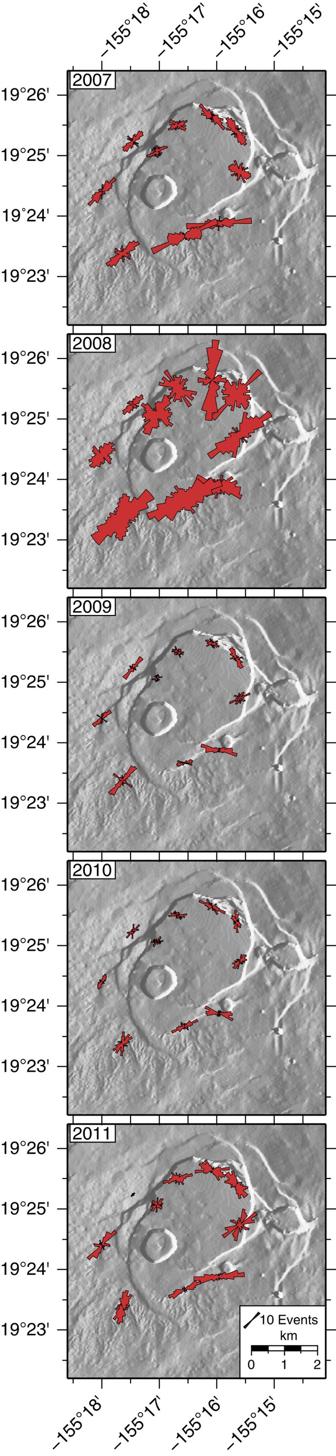Figure 2: Rose diagrams of the fast direction of anisotropy for each year. Rose diagrams (that is, circular histograms) plotted at the location of the recording station and scaled by number of measurements. A single, strong direction at each station, combined with the changes between closely spaced stations, suggests that the recorded anisotropy is acting directly beneath the station [3] . Stations within 1 km of significant faults (those that are large and shallow enough to have a surface expression) display structural anisotropy parallel to the faults. At the summit caldera, the background anisotropy is generally parallel to the caldera-bounding faults, suggesting that the anisotropy is usually caused by aligned fractures in the fault zones and is structurally controlled. Stations inside the caldera walls, however, display a change in ϕ , from parallel to the caldera walls in 2007, to radial to the caldera centre in 2008, and back to parallel in 2009 onwards ( Fig. 2 ). This change is particularly apparent and statistically significant in the north part of the caldera ( Fig. 1 , stations HAT, SBL and UWB), and less marked but still evident at stations closer to the vent ( Fig. 1 , stations BYL and OBL). 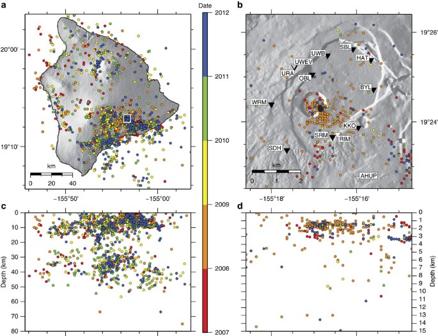Stations outside the main caldera-bounding faults do not display any temporal changes. Figure 1: Maps of the study area with earthquakes used in the analysis. Earthquakes are colour-coded by year of occurrence. (a) Map of the Island of Hawai‘i showing all earthquakes used in analysis (see text for selection criteria) and study region (white square). (b) Shaded-relief map of Kīlauea Caldera showing a subset of earthquakes and currently active vent (black ellipse). Black triangles indicate three-component seismometer stations, grey triangles indicate GPS stations used to obtain line length inFig. 3cand white triangle shows location of single-component seismometer used to obtain real-time seismic-amplitude measurement (RSAM) inFig. 3a. (c) Depth section across Hawai‘i Island west to east showing depth distribution of earthquakes. (d) Depth section across Kīlauea Caldera west to east showing shallow details of depth distribution of Caldera earthquakes. Figure 1: Maps of the study area with earthquakes used in the analysis. Earthquakes are colour-coded by year of occurrence. ( a ) Map of the Island of Hawai‘i showing all earthquakes used in analysis (see text for selection criteria) and study region (white square). ( b ) Shaded-relief map of Kīlauea Caldera showing a subset of earthquakes and currently active vent (black ellipse). Black triangles indicate three-component seismometer stations, grey triangles indicate GPS stations used to obtain line length in Fig. 3c and white triangle shows location of single-component seismometer used to obtain real-time seismic-amplitude measurement (RSAM) in Fig. 3a . ( c ) Depth section across Hawai‘i Island west to east showing depth distribution of earthquakes. ( d ) Depth section across Kīlauea Caldera west to east showing shallow details of depth distribution of Caldera earthquakes. Full size image Figure 2: Rose diagrams of the fast direction of anisotropy for each year. Rose diagrams (that is, circular histograms) plotted at the location of the recording station and scaled by number of measurements. Full size image SWS delay times There are no statistically significant variations in δ t at any of the stations ( Supplementary Fig. S1 and Supplementary Table S1 ). Although this result may seem surprising when considering the dramatic changes in ϕ within the caldera, small changes in the magnitude of anisotropy can create large variations in ϕ because ϕ and δ t are not coupled linearly, particularly when the mechanism of anisotropy varies [9] , [12] . At the times of the 2008 changes, therefore, subtle variations in δ t may be masked by scatter in the measurements [11] . The onset of Kīlauea's summit eruption in 2008 was not preceded by a dramatic change in the numbers of discrete earthquakes, nor by the usual inflationary ground deformation [16] , but SO 2 emissions ( Fig. 3b ) and seismic tremor ( Fig. 3a ) began to increase several months before the 19 March explosion [15] . SO 2 emissions increased from a background of ~150 tonnes per day in late 2007 to over 1500 tonnes per day before the eruption [17] , providing the most obvious indication of volcanic unrest and indicating a heightened rate of degassing of other magmatic volatiles, such as water. SO 2 emissions and seismic tremor have remained elevated throughout the course of the eruption, but both dropped when major vent collapses triggered week-long pauses in the eruption in December 2008 and again in mid 2009 ( Fig. 3a , solid grey bars) [14] . 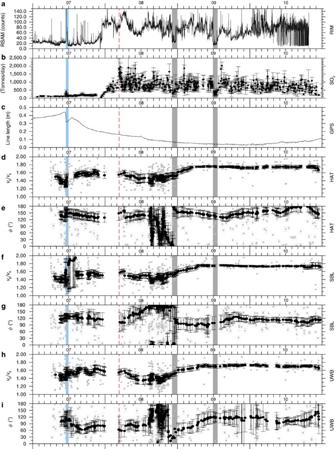Figure 3: Time series from January 2007 to December 2010. (a) RSAM recorded at seismic station RIM. (b) SO2emission rates at Kīlauea's summit17; vertical bars represent the s.d. for all traverses on a single day. (c) GPS line length between stations UWEV and AHUP. (d–i) SWSϕresults andVp/Vsat seismic stations in the north caldera. Grey points are individual measurements with error bars indicating 95% confidence interval, and black points are 30-point moving averages with error bars indicating the s.d. of the average. Solid blue vertical bar represents the Father's Day 2007 eruption, red dashed vertical bar marks the beginning of the summit eruption and solid grey vertical bars indicate pauses in the eruption. Figure 3: Time series from January 2007 to December 2010. ( a ) RSAM recorded at seismic station RIM. ( b ) SO 2 emission rates at Kīlauea's summit [17] ; vertical bars represent the s.d. for all traverses on a single day. ( c ) GPS line length between stations UWEV and AHUP. ( d – i ) SWS ϕ results and V p / V s at seismic stations in the north caldera. Grey points are individual measurements with error bars indicating 95% confidence interval, and black points are 30-point moving averages with error bars indicating the s.d. of the average. Solid blue vertical bar represents the Father's Day 2007 eruption, red dashed vertical bar marks the beginning of the summit eruption and solid grey vertical bars indicate pauses in the eruption. Full size image Variations in seismic anisotropy at Kīlauea's summit in 2008 may reflect changes associated with the formation of the summit eruptive vent between March and December 2008. The beginning of the shift in ϕ can be identified in the time series late 2007, coincident with the increase in both SO 2 emissions and tremor. Although deflating, pressure beneath the caldera remained high owing to the engorged nature of the magma system [16] , causing the maximum horizontal compressive stress to be radial. The increased gas pressure in shallow pore spaces opened more cracks parallel to the maximum horizontal compressive stress, changing the observed anisotropy to be radial to the caldera centre from late 2007 through 2008. This effect must be limited to the shallow subsurface because stations ~1 km apart display different ϕ . Because ϕ displays the direction of anisotropy from the last anisotropic media that the wave travelled through, it is reasonable that the anisotropy is acting at depths <1 km. Stations outside the caldera wall did not display the variation that those on the caldera floor exhibited, probably because the caldera floor is comprised of porous recent lava flows [18] , [19] . The state of stress inside the caldera, particularly that affected by the shallow (~1–2 km deep) magma reservoir, may be partially decoupled from outside the caldera due to the ring-fault system, which may also contribute to the lack of changes observed at stations on the caldera rim. The end of anomalous local SWS occurred in December 2008, at about the same time as a pause in the summit eruption (solid grey bar in Fig. 3 ). By this time, the new eruptive vent had stabilized and become the focal point of summit gas emissions (which were still high) as a direct pathway between degassing magma and the surface [20] . Gas was no longer fed into pore space in the shallow subsurface, causing pore pressure to return to background and SWS to return to its pre-eruptive, structurally governed state. Increased gas content in pores and cracks has the effect of lowering P-wave speed due to the higher fluid compressibility, but not significantly affecting the shear modulus, and hence S-wave speed. The ratio between P-wave velocity ( V p ) and S-wave velocity ( V s ), V p / V s , is therefore useful for characterizing pore-fluid content and supporting the SWS evidence. Laboratory measurements [21] show that crack opening induced by increasing pressure in gas-enriched pores leads to decreased V p / V s . Gas-enriched pore space has been reported to affect V p / V s above magmatic intrusions [22] , [23] , and several studies combine both SWS parameters and V p / V s to characterize pore content [13] , [24] . V p / V s was anomalously low (1.46±0.04) at Kīlauea in 2008 ( Fig. 3 ), after which it returned to a typical crustal value of 1.71±0.03 (ref. 25 ), supporting the hypothesis that the pore-gas content at shallow levels in the caldera was high in 2008. Use of catalogue origin times to calculate V p / V s will yield larger uncertainties (see the Methods section); however, if we take a V p / V s of 1.46, we can calculate a Poisson's ratio of ν =0.06, which is considerably lower than values previously observed ( ν =0.25–0.32) [26] . V p / V s after 2008 corresponds to ν =0.24, closely agreeing with previous investigators. V p / V s is sensitive to the entire ray path, and this is probably why all of the summit stations display a change in V p / V s rather than only the stations inside the caldera (the majority of the waves probably spend some time in the affected region). A small but similar deviation from background occurred in July 2007 ( Fig. 3 ). Although not a statistically significant change in ϕ or V p / V s , the presence of fluctuations in all of the time series and concurrence with the ‘Father's Day’ intrusion and eruption [16] suggests that the changes were driven by the same mechanism—degassing due to decompression of shallow magma [16] , increasing pore pressures and changing the seismic properties of the caldera. The Father's Day 2007 event was short-lived, allowing the system to quickly return to a background state and preventing strong SWS signals. Conversely, the onset of the summit eruption in 2008 and its continued activity was either prolonged enough or of a large enough magnitude to be reflected in the SWS signal, which returned to the background state only after the vent had become a well-established pathway for gas escape. SWS data presented here, when considered in isolation, could be consistent with the traditional interpretation of an inflating magma source subjecting the surrounding crust to a transient radial maximum horizontal compressive stress [8] . Ground deformation data showing deflation, however, do not support such a model. Combining SWS with V p / V s data allows us to conclude, instead, that the gas-filled pore pressure was high [13] at the start of Kīlauea's ongoing summit eruption—a model that is supported by high SO 2 emissions, which indicate increased rates of magmatic degassing. Although changes in SWS are traditionally interpreted as variations in the stress field [6] , we have shown that increased gas flux in volcanic areas may also create dramatic changes in SWS. Our results have two implications. First, changing SWS should not solely be interpreted in terms of stress conditions. Second, seismic observations could be used to infer changes in degassing from volcanic systems, which may be precursory to volcanic eruptions. These measurements may be carried out in near-real-time as a monitoring technique wherever earthquakes can be located and three-component seismometers are available. An advantage of this technique is that it is relatively insensitive to the seismicity distribution and does not rely on a dense network of seismometers, making it valuable at under-instrumented volcanoes. Shear wave splitting The algorithm for calculating SWS uses a grid-search inversion over the azimuth of the fast polarization direction ϕ and delay time δ t , for a given time window. It has been incorporated into code that conducts cluster analysis over a range of time windows to find the most stable result. The automated method [27] calculates the optimum three filters to apply to the data on the basis of signal-to-noise ratios and then determines the maximum and minimum time window around the S-wave arrival. These time window extremes are based on the dominant frequency of the first 3 s of the S-waveform. Uncertainties were calculated by finding the 95% confidence interval for the optimum values of ϕ and δ t after conducting an F-test for the chosen time window. The automated program was used to perform all SWS measurements in this study. The automated algorithm grades each measurement and marks any null measurements in which no splitting result is obtained. Results from the SWS analysis that gave ϕ to within 20 ° of the polarization of the incoming wave were considered null results. Nulls signify that no splitting was reliably detected, rendering the corresponding value of δ t meaningless and giving ϕ with a 90 ° ambiguity. The measurements were automatically graded based on signal-to-noise ratios and cluster characteristics. Only non-null results with a measurement grade of A or B and delay time <0.5 s were included. Measurements that differed substantially across filters were removed, and at most one measurement is presented for each earthquake-station pair. The incidence angle of each ray at each station is calculated using the TauP Toolkit [28] with the one-dimensional velocity model [29] for the Kīlauea region. In addition to the selection criteria enforced by the algorithm [27] , rays with incidence angles >35 ° from vertical were not included in the analyses as these lie outside the shear wave window, and S–P conversions at the surface could contaminate the waveforms. We observe that the steep velocity gradient in the top 0.5 km ensures that the majority of the local earthquakes that were recorded arrive at the stations with incidence angles <35 ° and so are included in the analysis. Significance of the changes in ϕ was tested by conducting a Rayleigh's test for the presence of a preferred trend ( Supplementary Methods , Supplementary Fig. S1 and Supplementary Table S1 ); where the 95% confidence intervals do not overlap, the change is significant. The changes were also tested by backazimuthal analysis to determine whether the variation is an artifact of changing earthquake location ( Supplementary Methods and Supplementary Fig. S2 ) and were found to be robust. V p /V s ratio The ratio of average P- to S-wave velocities is calculated following the approach of Nur [30] , using V p / V s = t s / t p with t s and t p representing the travel times of the S- and P-waves, which are calculated using catalogue locations and origin times. The average distance between seismic events and the stations they are recorded on is ~12 km. To preserve the S–P arrival time and account for the lower V p / V s ratio of 1.5, the hypocentral distance would have to increase by up to 5 km. The formal uncertainties in the catalogue locations are of the order of 800 m horizontally and 2 km vertically, and no change in earthquake location errors was detected during the time spanned; thus, the uncertainties on the locations cannot explain the change in V p / V s . The network configuration and methods of location have not changed over the timespan of this study, so it would be difficult (but not impossible) to explain the V p / V s variation as a systematic location error of up to 5 km. We therefore argue that the change in observed V p / V s ratio is caused by a decrease in V p and, although using the catalogue origin time to calculate t s and t p will yield a V p / V s ratio with larger uncertainties, we are confident that the trend in V p / V s is real. How to cite this article: Johnson, J. H. & Poland, M. P. Seismic detection of increased degassing before Kīlauea's 2008 summit explosion. Nat. Commun. 4:1668 doi: 10.1038/ncomms2703 (2013).